A freshwater predator hit twice by the effects of warming across trophic levels Many ecological responses to climate change have been documented. However, due to indirect effects, some responses can be complex and difficult to predict. For example, our understanding of effects on consumers involving responses on several trophic levels is limited. Here, combining the knowledge of trophic interactions in the EU’s fourth largest lake with long-term climate and catch data, we analyse potential drivers of change in this system’s apex predator. We show that warm winters correlate with later poor catches of great Arctic charr ( Salvelinus umbla ), and that in recent years predator–prey cycles involving this species have disappeared. The likely mechanisms are trophic mismatches directly and indirectly affecting two stages of charr, the fry and the juveniles, respectively. Our study illustrates how a long-lived consumer may be subjected to double jeopardy from the effects of warming across trophic levels, and that a food web approach can aid in disentangling the chain of mechanisms responsible. Studies show that climate is changing globally, regionally as well as locally [1] , and ecological responses to climate change have been documented across many levels of biological organization and different types of ecosystems [2] , [3] , [4] , [5] . As a result, together with habitat change and introductions of non-native species, climate change now represents an important and increasing threat to species as well as the structure and functioning of ecosystems [6] , [7] , [8] . Climate change not only causes comparably simple, direct (physiological) responses of species, but may also lead to indirect effects [4] , for example, by affecting interactions between species [9] , [10] . This may occur if interacting species show differential physiological or behavioural responses to climate change [11] , [12] leading to, for example, changes in competitive dominance between species [13] , or trophic mismatches [14] , [15] between consumers and their resources. Such indirect effects to warming have been documented in both marine and terrestrial systems [11] , [16] . However, because some indirect effects may involve more than two species, and species may react to primary, as well as secondary responses of other species, ecological effects of warming can be very complex and difficult to predict [17] and could potentially cascade through an entire community [18] . As a result, our understanding of effects on species involving responses on several trophic levels is yet limited. Freshwater ecosystems—being comparably well defined and closed systems where many species spend their entire life cycle—could be good model systems to address this deficit and study effects of warming across trophic levels. Although examples of direct responses to climate change in freshwater systems are mounting [5] , [19] , [20] , [21] , [22] , much of our understanding of warming effects in these systems, including a few cases of documented trophic mismatches [23] , [24] , [25] , [26] , is based on studies of plankton communities (for example, showing increased abundance of small-sized phytoplankton species [19] , [27] , [28] , increasing cyanobacteria abundance [20] , [21] , [29] , [30] and shifts in the zooplankton community structure [22] , [31] ), while indirect effects across trophic levels on higher level consumers are much less studied [5] . In fact, we know of no example of indirect effects of climate change on an apex predator in a freshwater system where the mechanisms operating across trophic levels have been analysed. Furthermore, a pressing issue is how populations that already are endangered, due to other anthropogenic stressors, will respond to a combination of direct and indirect effects of climate change and how their management may need to be adjusted [32] . This is particularly true for many aquatic species that may have less potential for dispersal in response to a changing climate (when compared with many marine or terrestrial species). Here we address these issues by analysing the climate effects on an endangered [33] stock of Arctic charr (great Arctic charr; Salvelinus umbla )—the apex predator in the second largest lake in Sweden (Lake Vättern, Supplementary Fig. 1 )—to study the effects of warming across multiple trophic levels and be able to discuss implications of this for future climate change effects on the population. Since species within the Arctic charr complex in general are considered sensitive to climate change [34] , an increased understanding of how warming could affect the stock of great Arctic charr in Lake Vättern can have broader implications for similar species in other ecosystems. Disentangling the possibly complex mechanisms driving the effects of warming on a population hinges on the identification of critical stages in the life cycle and knowledge of important interactions with other species and how these may be affected by climate. Here this analysis is aided by a good understanding of the trophic interactions in the pelagic food web of Lake Vättern and the ontogenetic niche shifts in its apex predator ( Fig. 1 ). Using a combination of data on commercial catches, and environmental data, we analyse whether warming has affected three potentially critical life stages of Arctic charr—the fry, small juveniles and large juveniles—via effects on availability of their main food: zooplankton, crustaceans and vendace ( Coregonus alba ). We show that winter water temperature has a time-lagged effect on (normalized) catches of charr, with warm winters being correlated with poor catches of great Arctic charr 5–6 years later, and the last 25 years of warming has seen the disappearance of closely linked predator–prey cycles involving charr and one of its main prey species, vendace. We argue that the likely mechanisms in both cases are trophic mismatches [11] , [15] , [16] affecting two different life stages of Arctic charr, the first acting directly on fry of Arctic charr and the other indirectly on a later stage, via another species. Our study illustrates how a long-lived consumer may be subjected to a double jeopardy from the effects of warming across trophic levels and how a food web approach can aid in disentangling the chain of mechanisms responsible. 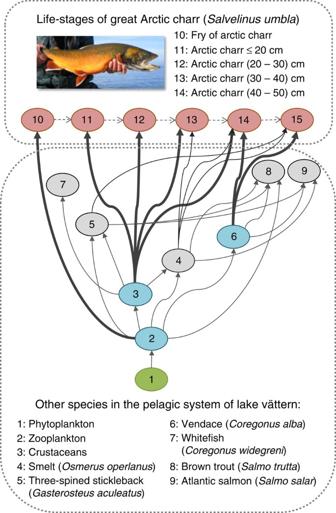Figure 1: The pelagic food web of Lake Vättern. Dashed arrows: development between stages of Arctic charr (red nodes). Solid arrows: trophic links. Potentially important resources and trophic links for Arctic charr that are studied here are denoted by turquois nodes and thick solid arrows. Green and grey nodes, respectively, represent the primary producers in the system and species not studied here. The structure of the food web is based on stomach content analyses46,53. Figure 1: The pelagic food web of Lake Vättern. Dashed arrows: development between stages of Arctic charr (red nodes). Solid arrows: trophic links. Potentially important resources and trophic links for Arctic charr that are studied here are denoted by turquois nodes and thick solid arrows. Green and grey nodes, respectively, represent the primary producers in the system and species not studied here. The structure of the food web is based on stomach content analyses [46] , [53] . Full size image Commercial catch and survey data The fishery data for Arctic charr show an initial trend of increasing catches, but after peak catches during 1930–1950, ever decreasing amounts until record lows in recent years ( Fig. 2a ). Catches of vendace peak in the 1960s, after which they dwindle ( Fig. 2b ). Survey data indicate that the abundance of crustaceans has fluctuated since 1971 ( Fig. 2c ), but without any clear trend. Spectral power analyses show that original time series of both vendace and charr ( Supplementary Fig. 2a,d ) are dominated by very long period (low-frequency) fluctuations (>30 years). As the time series are normalized (using a trend line to reduce long-term changes in catch effort and efficiency, see Methods), these very long period fluctuations are lost, producing time series with a flat power spectrum ( Supplementary Fig. 3 , indicating detrended time series where variation on no timescale dominates). 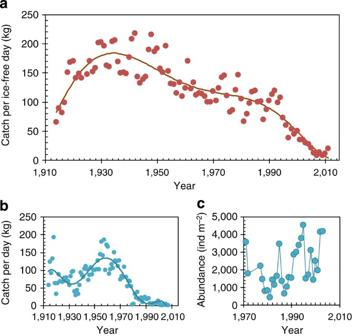Figure 2: Fishery catch data and survey data on crustaceans in Lake Vättern. (a) Commercial catches of Arctic charr (red filled circles); (b) commercial catches of vendace (turquois filled circles); (c) survey abundances of crustaceans (turquois filled circles). Solid lines ina,bare fitted polynomial trendlines (a):R2=0.84, F-test:P=7.2·10−31,n=97, (b):R2=0.79, F-test:P=1.6·10−23,n=97) used to normalize the observed catch data. Figure 2: Fishery catch data and survey data on crustaceans in Lake Vättern. ( a ) Commercial catches of Arctic charr (red filled circles); ( b ) commercial catches of vendace (turquois filled circles); ( c ) survey abundances of crustaceans (turquois filled circles). Solid lines in a , b are fitted polynomial trendlines ( a ): R 2 =0.84, F-test: P =7.2·10 −31 , n =97, ( b ): R 2 =0.79, F-test: P =1.6·10 −23 , n =97) used to normalize the observed catch data. Full size image Arctic charr versus water temperature and zooplankton Until around 1990, water temperature fluctuated ( Fig. 3a ) but without any significant trend. A segmented regression analysis yields a breakpoint in 1986, with the period after this showing a significant increase in yearly mean water temperature ( Fig. 3a ). Similar results are found for both winter and spring water temperature (months November to March, Supplementary Fig. 4a–f ), but with the breakpoint varying between 1982 and 1996 (with 1990 being the average year). Interestingly, the effect is strongest (steepest slope) for winter months (November–February) and weakest for spring months March and April. For late spring (May), no significant trend in water temperature could be found ( Supplementary Fig. 4g ). 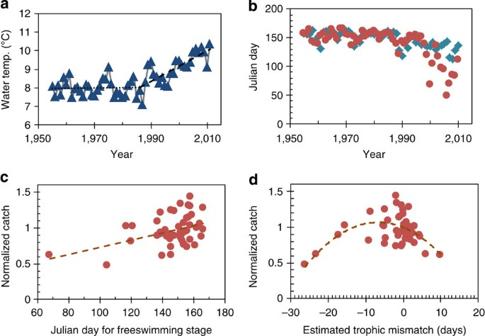Figure 3: Relation between water temperature, fry and plankton phenology and catches of Arctic charr in Lake Vättern. (a) Yearly mean water temperature based on daily measures (dotted and dashed lines are least-squares regression lines of segmented linear regression, yielding a breakpoint at 1986 and a non-significant and significant (F-test:P<0.001) slope of the first (n=32) and second (n=26) segment, respectively); (b) Predicted ordinal dates for reaching the free-swimming stage of fry of great Arctic charr (red circles) and spring peak in plankton abundance (turquois diamonds) using winter and spring water temperature data, respectively; (c) Relationship between normalized catch of charr and the date when fry are predicted to become actively foraging 5 years earlier; (d) Relationship between normalized catch and the estimated trophic mismatch between fry and zooplankton. Dashed lines inc,dare least-squares linear (c):R2=0.17, F-test:P=0.0035,n=49) and quadratic (d):R2=0.35, F-test:P=0.00019,n=49) regression lines (quadratic regression indyielded a significantly better fit than a linear model F-test:P=0.0000013). Figure 3: Relation between water temperature, fry and plankton phenology and catches of Arctic charr in Lake Vättern. ( a ) Yearly mean water temperature based on daily measures (dotted and dashed lines are least-squares regression lines of segmented linear regression, yielding a breakpoint at 1986 and a non-significant and significant (F-test: P <0.001) slope of the first ( n =32) and second ( n =26) segment, respectively); ( b ) Predicted ordinal dates for reaching the free-swimming stage of fry of great Arctic charr (red circles) and spring peak in plankton abundance (turquois diamonds) using winter and spring water temperature data, respectively; ( c ) Relationship between normalized catch of charr and the date when fry are predicted to become actively foraging 5 years earlier; ( d ) Relationship between normalized catch and the estimated trophic mismatch between fry and zooplankton. Dashed lines in c , d are least-squares linear ( c ): R 2 =0.17, F-test: P =0.0035, n =49) and quadratic ( d ): R 2 =0.35, F-test: P =0.00019, n =49) regression lines (quadratic regression in d yielded a significantly better fit than a linear model F-test: P =0.0000013). Full size image Before 1990, the predicted date for the larvae of Arctic charr to reach the actively foraging fry stage varied ( Fig. 3b ), but was, on average, well matched to the estimated timing of the zooplankton peak. However, around 1990, increasing water temperatures causes the dates for both fry and zooplankton to advance. This trend is much stronger for the fry though, leading to a developing gap between the dates for reaching the free-swimming stage and the predicted zooplankton peak. Furthermore, our data show that early dates for the fry to emerge are significantly associated with smaller normalized catches, 5 ( Fig. 3c ), 6 as well as 7 years later (F-test: P =0.0035, n =49; P =0.0041, n =48 and P =0.047, n =47, respectively), when those fry have grown and are expected to dominate the catch ( Supplementary Fig. 5a ). For slightly shorter and longer time lags, there are also positive, but non-significant correlations between catch and date for reaching the free-swimming stage (F-test: P =0.13, n =50 and P =0.22, n =47 for time lags of 4 and 8 years, respectively). Finally, when taking the predicted date for reaching the free-swimming stage relative to the zooplankton peak into account, we find a significant quadratic relationship (F-test: P =0.00019, n =43, Fig. 3d ) between normalized catches of Arctic charr and the estimated degree of trophic mismatch that has affected the catch in a particular year (see Methods). This relationship explains twice the amount of variation in catches compared with if the expected date for the zooplankton peak is not taken into account ( Fig. 3c ). Arctic charr versus water temperature and vendace Spectral analysis of normalized (detrended) time series of both charr and vendace ( Supplementary Fig. 2 ) indicate the presence and dominance of fluctuations with a period of 4–8 years before significant warming (determined by breakpoint in Fig. 3a ), but not after. Furthermore, before, but not after, this divide, detrended time series of both Arctic charr and vendace show significant negative autocorrelations at a time lag of 3 years ( Fig. 4a,c ; indicating cycles with a period of ~6 years). That these cycles are coupled is supported by the cross-correlation function ( Fig. 4b,d ), showing that catches of Arctic charr are positively correlated to catches of vendace 2 years earlier, and negatively to catches of vendace 1 year later (also suggesting cycles with an amplitude of ~6 years). In line with the indication that the time series of vendace and Arctic charr are linked, we see a tendency for rotation of the trajectories of both species in phase space ( Fig. 5 ). More specifically, breaking up the study period into shorter time intervals (with a length that varies between 4 and 8 years, corresponding to the range of periods indicated by the spectral analysis, Supplementary Fig. 2 ) illustrates a dominance of counter-clockwise rotation before significant warming, with 9 of the 11 first time intervals showing indication of counter-clockwise rotation. Four of the five intervals since 1985 instead produce more or less random trajectories in phase space, with no obvious cyclic pattern. 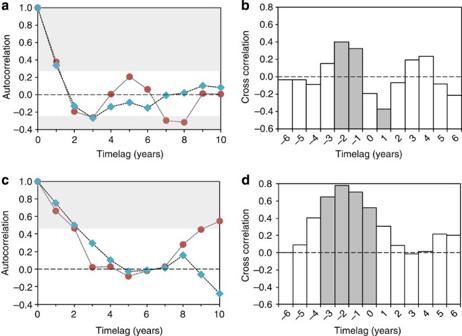Figure 4: Autocorrelation and cross-correlation of normalized time series of great Arctic charr and vendace in Lake Vättern. (a) The autocorrelation function of normalized time series of great Arctic charr (red circles) and vendace (turquois diamonds) before 1986. (b) The cross-correlation between normalized time series of great Arctic charr and vendace before 1986. (c) The autocorrelation function of normalized time series of great Arctic charr (red circles) and vendace (turquois diamonds) after 1986. (d) The cross-correlation between normalized time series of great Arctic charr and vendace after 1986. Data points in shaded regions ina,cand shaded bars inb,drepresent the correlations that deviate significantly (F-test) from zero (dashed line) atP<0.05. Figure 4: Autocorrelation and cross-correlation of normalized time series of great Arctic charr and vendace in Lake Vättern. ( a ) The autocorrelation function of normalized time series of great Arctic charr (red circles) and vendace (turquois diamonds) before 1986. ( b ) The cross-correlation between normalized time series of great Arctic charr and vendace before 1986. ( c ) The autocorrelation function of normalized time series of great Arctic charr (red circles) and vendace (turquois diamonds) after 1986. ( d ) The cross-correlation between normalized time series of great Arctic charr and vendace after 1986. Data points in shaded regions in a , c and shaded bars in b , d represent the correlations that deviate significantly (F-test) from zero (dashed line) at P <0.05. 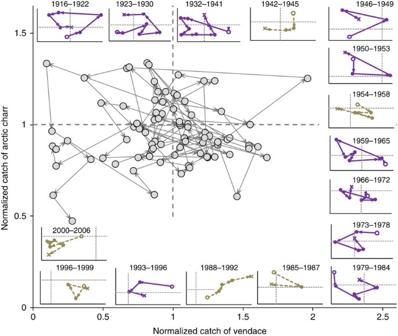Figure 5: Phase space portraits of population dynamics of great Arctic charr and vendace in Lake Vättern through time. Combinations of normalized catches of vendace and great Arctic charr for the entire study period are depicted by grey circles in the main plot area. Inserts separately plot time periods during which there is (purple markers and solid lines), or is not (light brown markers and dashed lines), indication of a counter-clockwise evolution of catches. The starting point for every trajectory is indicated by an open circle and the end point by a cross. Note that length of time periods differ and axes scales of inserts are not identical, but have been modified for best visualization of trajectories. Full size image Figure 5: Phase space portraits of population dynamics of great Arctic charr and vendace in Lake Vättern through time. Combinations of normalized catches of vendace and great Arctic charr for the entire study period are depicted by grey circles in the main plot area. Inserts separately plot time periods during which there is (purple markers and solid lines), or is not (light brown markers and dashed lines), indication of a counter-clockwise evolution of catches. The starting point for every trajectory is indicated by an open circle and the end point by a cross. Note that length of time periods differ and axes scales of inserts are not identical, but have been modified for best visualization of trajectories. Full size image Finally, the trophic control indices (indicating positive and negative correlations between time series of vendace and Arctic charr on shorter timescales than the cross-correlation function) show simultaneous bottom–up and top–down control between vendace and Arctic charr for most of the study period ( Fig. 6a ). Before 1990, the only exception occurs around 1940 (corresponding to the one exception to counter-clockwise rotation in phase space before 1984). Starting around 1990, however, and significantly correlated to an observed increase in winter water temperatures ( Fig. 6b ), the concurrent bottom–up and top–down control gradually disappear (F-test of correlation between bottom–up and top–down indices and winter water temperature: R =−0.72, P <0.001, n =49 and R =0.52, P <0.001, n =49 respectively). 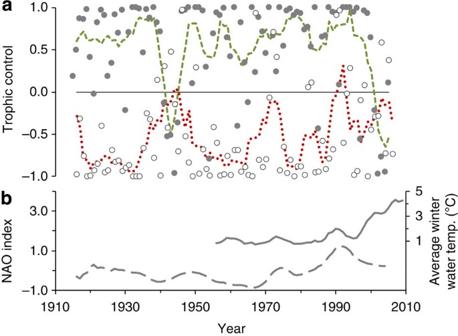Figure 6: Relation between population dynamics of great Arctic charr and vendace in Lake Vättern through time and in relation to warming. (a) variation over time in the degree of top–down (red dotted line, open circles) and bottom–up (green dashed line, shaded circles) control between great Arctic charr and vendace; (b) Variation over time in the NAO winter index (grey dashed line) and average winter (December through March) water temperature (solid grey line). The trophic control indices inashow the correlations between catches of great Arctic charr and vendace on a sliding time window (shaded and open circles) from which 5-year running means (green and red dashed lines) were calculated. NAO PC-based winter (January through March) index data70were obtained from the Climate Analysis Section, NCAR, Boulder, USA71. Figure 6: Relation between population dynamics of great Arctic charr and vendace in Lake Vättern through time and in relation to warming. ( a ) variation over time in the degree of top–down (red dotted line, open circles) and bottom–up (green dashed line, shaded circles) control between great Arctic charr and vendace; ( b ) Variation over time in the NAO winter index (grey dashed line) and average winter (December through March) water temperature (solid grey line). The trophic control indices in a show the correlations between catches of great Arctic charr and vendace on a sliding time window (shaded and open circles) from which 5-year running means (green and red dashed lines) were calculated. NAO PC-based winter (January through March) index data [70] were obtained from the Climate Analysis Section, NCAR, Boulder, USA [71] . Full size image Arctic charr versus water temperature and crustaceans For glacial relict crustaceans, we find only marginally significant autocorrelations at time lags of 4 and 5 years (F-test: P =0.085, n =23 and P =0.080, n =22 respectively). Furthermore, cross-correlation analysis of the time series show a significant positive correlation (F-test: P =0.025, n =26) between the biomass abundance of crustaceans in one year and the relative catch of Arctic charr 1 year later. Time series of Arctic charr and crustaceans, however, produce a more or less random trajectory in phase space, with no obvious cyclic pattern and the trophic control indices show no sign of any decreasing trend since 1990 or any correlation with winter water temperature ( Supplementary Fig. 6 ), suggesting no effect of warming on the interaction between crustaceans and Arctic charr. Finally, the slope of the power spectra is significantly negative for crustaceans (F-test: P =0.0022, n =15), suggesting a slight redshift in the population dynamics of glacial relict crustaceans that is seen in neither vendace nor Arctic charr. Here we have analysed the potential effects of climate on great Arctic charr, the apex predator in Lake Vättern, the second largest freshwater system in Sweden. Our data indicate that warming has affected two out of three potentially critical life stages of Arctic charr (the fry, small juveniles and large juveniles, Fig. 1 ), via the effects on availability of their main food (zooplankton and vendace). This suggests that warming during recent decades—in addition to other factors such as overharvesting and introduced species [35] that may have been responsible for initiating and driving the first phase of the downward trend in the stock of Arctic charr ( Fig. 2 )—has become an additional and maybe increasingly important stressor on Arctic charr, which needs to be considered in the management of the species. More specifically, we show that some sort of regime shift appears to have occurred in Lake Vättern around 1990, when suddenly increasing water temperatures coincide with both smaller than expected catches of Arctic charr and changed population dynamics. What could the mechanisms behind these observations be? To begin with, water temperature affects both the developmental rate of eggs of Arctic charr and the timing of the zooplankton peak. Thus, we see that when water temperatures start to increase ( Fig. 3a ), this causes the dates for both fry to reach the free-swimming stage and zooplankton to advance ( Fig. 3b ). However, because the developmental rate of eggs is dependent on winter water temperature (spawning occurs in late October), while the timing of the zooplankton peak mainly is determined by spring water conditions, and the increase in water temperature is stronger for winter months (November–February, Supplementary Fig. 4a–d ) than for spring months (March and April, Supplementary Fig. 4e,f ), the advancing trend is much stronger for the fry than for zooplankton ( Fig. 3b ). This suggests that recruitment to the stock of Arctic charr could be negatively affected by a developing trophic mismatch [14] , [15] due to the fry emerging at a time of suboptimal resource abundance. Although we acknowledge that truly independent data do not exist for this interpretation, it is supported by two related observations. First, if increasing water temperatures are affecting the stock of Arctic charr negatively, via a trophic mismatch, years with warm winter temperatures (that result in early hatching and presumably poor recruitment) could be expected to affect catches of charr, but with some time lag depending on the time it takes for fry to grow into the catch. This is exactly what we find ( Fig. 3c ). Because the effect is significant at a time lag of 5 to 6 years, and this corresponds to the time needed for newly hatched fry to grow to a size when they are expected to dominate the catch ( Supplementary Fig. 5 ), we have strong reasons to believe that warming actually is affecting the survival of fry, via food availability during the critical free-swimming stage. Indeed, lending further support to this interpretation, we find that the greater the predicted contribution of an age class j to the total catch ( Supplementary Fig. 5 ), the stronger we find the association to be between catches and the date ( j years earlier) that the fry of that age class emerged ( R =0.83, F-test: P =0.0026, n =10). In other words, our data suggest a trophic mismatch, where temperature affects both the development rate of charr eggs (and thus time of reaching the free-swimming stage of fry) and the availability of food resources for the fry. Second, according to the trophic mismatch hypothesis [15] , ‘success’ of a consumer (survival and/or reproduction) depends on the timing of the consumer relative to the peak in prey abundance [11] , suggesting here that both early and late dates to reach the free-swimming stage, relative to the zooplankton peak, could result in smaller than expected catches. To be able to explore this possibility, we needed to predict the timing of peak zooplankton abundance and interestingly, we find consumer success (here indicated by normalized catches of charr) to be related to the estimated mismatch in timing between consumer and resource exactly as predicted by theory [16] (but to our knowledge never shown empirically). To summarize, these data are strong support for the existence of a trophic mismatch between the fry of Arctic charr and zooplankton. To further disentangle the complex mechanisms driving the effects of climate on populations and ecological communities, it can be informative to study how warming modifies the strength of trophic relationships, particularly those involving potential keystone species [36] , [37] , [38] , [39] and that may affect the population dynamics of other species and relative importance of top–down and bottom–up forces in communities [40] , [41] , [42] . In our system, vendace is an important link between the base and top of the pelagic food web, due to its role as both a significant zooplankton consumer and an important prey species for the apex predator ( Fig. 1 ), making it a potential keystone species that could mediate external forcing, such as climate effects, between different parts of the food web and affect the population dynamics of species. In support of a strong link between vendace and Arctic charr, we found the time series of these species to be associated for a long time ( Fig. 4b,d ), with a tendency for cyclic behaviour ( Fig. 4a,b and Supplementary Fig. 2 ) and dominance of a pattern characteristic of classical predator–prey cycles ( Figs 5 and 6 ). These characteristics of the association between vendace and charr appear to change around 1990, however, as winter water temperatures start to increase significantly, raising the possibility that vendace could be a mediator of climatic effects from lower trophic levels with warming leading to a decrease in the importance of vendace for charr. In support of this interpretation, other studies [43] , [44] indicate that vendace dynamics in the great lakes of Sweden are affected by (at least) four factors. First, because vendace is zooplanktivorous during its entire life, there is asymmetric intraspecific competition between adults and juveniles, where strong year classes can dominate the stock for several years and prevent successful recruitment [43] . Such strong year classes either have to ‘die away’ due to natural mortality, or be reduced by predation, before a new pulse of successful recruitment can occur. Our analyses (indicating significant top–down control of charr on vendace, Fig. 4b,d and Fig. 6 ) suggest that predation from Arctic charr may have been partly responsible for this. Second, ice winters with late ice break-up have been associated with favourable plankton conditions in the great lakes and as a consequence high recruitment rates and later strong year classes in vendace [43] . This suggests that warming will affect vendace negatively by leading to fewer winters with ice and earlier ice break-up. Third, since vendace, like Arctic charr, is an autumn spawner, winter water temperature will also have a direct physiological effect on vendace, in the same way as on charr (leading to faster development of eggs), suggesting that warming could affect vendace negatively also by its effect on the timing of emergence of fry in the spring. We do not have the data necessary to predict hatching of eggs of vendace in Lake Vättern (as we did for great Arctic charr), but we do find a significant negative correlation (F-test: P =0.0068, n =49) between winter (December through March) water temperature and catches of vendace 2 years later, which strongly support the hypothesis that recruitment in vendace is affected by winter water temperature, possibly due to a trophic mismatch. Finally, smelt ( Osmerus operlanus ) is a spring spawner and a competitor with vendace for zooplankton ( Fig. 1 ), and a warmer climate has been associated with positive effects on growth rates [45] and recruitment [44] of smelt in oligotrophic deep-water lakes. This means that vendace and smelt could be responding differently to a warmer climate and, as a consequence, that the importance of vendace, relative to smelt, as a prey for Arctic charr could change. This indeed seems to be the case for Arctic charr in the size class 40–49 cm, where the proportion of smelt over the last 30 years [46] has increased (from ~50% to ~90%, and vendace decreased (from ~35% to ~15%). Taken together, all this suggests that warming since 1990, in combination with an already depleted stock of Arctic charr, has disrupted the strong link between vendace and charr, with (i) warmer winters leading to fewer years favourable for recruitment of both species and stronger competition between vendace and smelt and (ii) Arctic charr being less able to initiate a downward trend in the less frequently occurring strong year classes of vendace. The result is a stock of vendace with reduced average abundance and longer period of fluctuations (as seen in recent analysis of survey data in Lake Vättern [44] ) and a stock of great Arctic charr that no longer fluctuates in synchrony with vendace. In Europe, many populations of Arctic charr have declined [47] , [48] , with many declines being, at least partly, linked to climate change [48] , [49] . Considering this and the effects of warmer winters we have uncovered here, an important question is what will happen to the endangered stock of great Arctic charr in Lake Vättern, if warming continues as predicted. Adapting to a changing environment involves either plastic responses, or genetic change, the relative importance of which are debated [50] . With respect to the trophic mismatch discussed here, adaptation would involve adjusting the date for spawning in the fall and/or developmental rate of the eggs. The negative effects of warming we have observed indicate that plasticity in these traits either is absent or insufficient to close the mismatch gap between the fry and zooplankton, implying that genetic change is necessary. However, genetic change hinges on genetic variability, which in turn is related to population size. Thus—since any action to reduce climate change will be slow to take effect and measures so far have been insufficient to stop further warming—the best way to help great Arctic charr cope with climate change is probably to avoid a further population decrease, and instead help the stock to increase in abundance, so that adaptation becomes more feasible. This objective is particularly pressing considering that today a suite of stressors, in addition to warming, are affecting the population. These include predation on eggs by introduced crayfish [35] , competition from introduced salmon and commercial and recreational fishing. Thus, somewhat counterintuitive, our study suggests that taking the threat from warming seriously implies that the future management of great Arctic charr will need a focus on reducing these additional stressors. To conclude, in northern regions, a warmer climate can be expected to decrease cold stress in winter [51] and increase growth rates in summer, suggesting a simple positive effect on many species, all else being constant. However, in most cases, direct and indirect interactions with other species also are likely to change. This calls for a food web-oriented approach to study the net effects of climate change on species, which due to indirect effects could be opposite in sign from the direct effects. The mechanisms responsible for the effects of warming documented here operate across several trophic levels, involving primary, secondary as well as tertiary responses of an apex predator to perturbations from climate change. Primary responses comprise effects of winter water temperature on (i) the spring peak of zooplankton and (ii) the developmental rate of eggs of vendace and great Arctic charr. Secondary responses include the dwindling recruitments to the stocks of both vendace and Arctic charr, which result from differential primary responses of consumers and prey (that is, with the date for reaching the actively foraging stage of fry advancing faster than the date of the zooplankton spring peak). Although definitely important, such primary and secondary responses to warming have been documented before and the mechanisms involved are fairly straightforward. However, tertiary responses, involving the response of one species to the secondary response of another species, are less studied and the mechanisms could be challenging to disentangle. Here we infer the existence of such a tertiary response, with great Arctic charr responding to the secondary response to warming of one of its prey (vendace). The net results are changed population dynamics and a negative effect on the stock of Arctic charr mediated via the negative effect of warming on vendace. This scenario implies an interesting, but previously unrecognized, possibility: a long-lived consumer, wherein the individuals display ontogenetic niche shifts, may be subjected to the negative effects of a particular phenological change twice. This double jeopardy from climate change can occur if an early life stage of the consumer shares resources with a species that is also a prey of a later life stage (of the consumer) and a similar trophic mismatch is affecting both species. If correct, this means that increasing winter water temperature will affect Arctic charr negatively, firstly via a trophic mismatch between its own fry and zooplankton, and secondly via decreasing abundance of vendace (caused by a second trophic mismatch between fry of vendace and zooplankton). We anticipate that many more similar tertiary, or even quaternary, effects are present in other systems, waiting to be unravelled using a food web approach, so that our understanding of warming across multiple scales and levels of organization [5] can be increased. Study system and organisms Lake Vättern, Europe’s sixth largest lake, is a deep, oligotrophic lake in south-central Sweden ( Supplementary Fig. 1 ) that harbours some 30 species of fish, among these a unique, large-bodied, non-anadromous form of Arctic charr (great Arctic charr). This species is the largest naturally occurring predator in Lake Vättern. Historically, this population was important for commercial fishing, but the stock has decreased considerably in size during the second part of the twentieth century [52] , causing it to be red-listed as critically endangered [33] . Causes for the collapse are debated, with the main competing hypotheses being overharvesting, introduced species, reduced nutrient loading and climate change [46] . Predation on eggs of charr by alien signal crayfish ( Pacifastacus leniusculus ) was recently studied experimentally and found to be potentially significant [35] . The focus of this contribution is on the potential effects of warming. Great Arctic charr matures late and can reach an age of up to 25 years, weigh up to 11 kg and reach a length of 85 cm. Spawning takes place in the fall with development time of eggs, and thus time of hatching, dependent on winter water temperature. Newly hatched larvae are initially inactive and live on yolk for a short period, before starting to forage actively as they reach the fry stage. Stomach content analyses [46] , [53] , [54] , [55] have resulted in a well-resolved view of the feeding relations in the off-shore part of Lake Vättern, especially with regard to great Arctic charr ( Fig. 1 ). The fry feeds on zooplankton, before focusing on crustaceans (mainly Mysis relicta , Monoporeia affinis and Pallasea quadrispinosa ) as small juveniles in the size interval 10–20 cm [53] . As the individuals grow, they gradually switch to a fish diet, first dominated by smelt when in the size interval 30–40 cm, via a mix of vendace, smelt and three-spined stickleback ( Gasterosteus aculeatus ) when in the size interval 40–60 cm, to a dominance of vendace when >60 cm (refs 46 , 53 ). This suggests that there are several potentially important phases in the life cycle, where prey abundance and/or climate could affect survival, and subsequently (with some time lag, depending on the growth rate of the fish and size regulation of the fishery) the size of the stock available to the fishery. Water temperature data and data on ice cover Daily water temperature data for the period 1955–2011 come from the northern part of Lake Vättern (by the outlet into the river Motala ström) and were provided by the County Administrative Board in Jönköping. For some days, data were missing and the water temperature for these days (4.7% of winter days, from spawning in the fall to May, during the study period) were estimated by linear interpolation between the preceding and following days with data. From these daily data, a moving 3-day average water temperature was calculated for each day to reduce daily random variability in water temperature (due to measurement error and so on). Because winters with ice may affect fishing (see below), data on formation, break-up and duration of ice cover on Lake Vättern 1914–2011 ( Supplementary Table 1 ) was obtained by merging two sources: ref. 56 for the period 1914–1961, and data from the County Administrative Board for the period 1962–2011. Lake Vättern is a deep, long and narrow lake where strong winds during winter affect ice formation negatively so that the lake very seldom is completely covered by ice. Ice cover on the lake was here defined as when there was ice between the island Visingsö and the mainland on the eastern shore (see Supplementary Fig. 1 ). When this part of the lake freezes, most of the lake tends to be covered by ice. Fishery catch data and survey data on crustaceans Detailed stock survey data of great Arctic charr, and other pelagic fish species in Lake Vättern, are only available for a few recent years (2006–2011). Instead, indirect indications of stock abundance were needed to analyse the effect of climate on Arctic charr on a longer time perspective. Commercial catch data (tons per year) for vendace and Arctic charr is available since 1914, but without any description on how effort and efficiency in the fishery have varied. Thus, to reduce the effect of long-term trends in effort, efficiency and stock abundance on the catch and focus on variability in catch that could indicate variation in stock size due to climate, we normalized the catch data—in the case of Arctic charr corrected for a significant effect of days available for fishing due to winters with ice ( Supplementary Table 1 )—relative to a trend line. More specifically, we fitted polynomial functions ( , where E(X) is the predicted catch in year X ) of increasing order ( n =1, 2, …10) to the observed catches of vendace (kg per day) and Arctic charr (kg per ice-free day). Polynomial trendlines of order four and higher all resulted in a high level of explained total variability ( R 2 >0.8 for Arctic charr and R 2 >0.73 for vendace, Supplementary Fig. 3a,b ). We then used power spectral analysis to decompose the remaining (unexplained) variability into variation on different timescales and looked for trendlines with a flat power spectrum of residuals, indicating a detrended time series where variation on no timescale dominates. The original time series of observed (that is, non-normalized) catches of Arctic charr and vendace were both significantly redshifted (slope=−1.70, F-test: P <0.001 and slope=−0.91, F-test: P =0.02, respectively). Polynomial trendlines captured first long-term (low-frequency) variability, and with increasing order also more and more of the intermediate-term, and then short-term (high frequency) variability. This translated to a gradual change in the slope of the power spectrum of residuals ( Supplementary Fig. 3c,d ), from initially negative (with too little of the long-term variability captured), to a positive slope (with only very short-term variability remaining). The target criterion of a more or less flat power spectrum, was fulfilled for polynomial trendlines of orders five to seven for Arctic charr and five to six for vendace ( Supplementary Fig. 3c,d ). In all subsequent analyses, and results presented in our study, the normalized catches ( ρ X ) of both Arctic charr and vendace are based on order six polynomial functions and was calculated as: (where O X is the observed catch in year X and E(X) is the predicted catch in year X according to the trend line). However, results and conclusions presented here are not dependent on using the order six polynomial, since using polynomial functions of order five, six and seven (all with a flat power spectrum of residuals) resulted in trendlines that produced qualitatively similar results. Macroinvertebrate data have been collected in late summer at two sampling stations in Lake Vättern ( Supplementary Fig. 1 ) between 1971 and 2003, as part of a national environmental monitoring programme [57] . We used the average of the two stations late summer profundal sample biomass abundance of Malacostraca ( Mysis relicta , Monoporeia affinis , Relictacanthus lacustris , Pallasea quadrispinosa and Saduria entomon ; sampling depth 60–100 m) to test for the effects of abundance of crustaceans on great Arctic charr. Predicted time for fry to reach free-swimming stage Spawning time for great Arctic charr in Lake Vättern is temporally more or less constant with 20 October as the median date when spawning activity peaks. The eggs hatch after ~485 ° C degree days [58] (accumulated daily water temperatures), usually in late winter/early spring. Much of the yolk sac of the larvae is consumed after ~750 ° C degree days, and the larvae reaches the free-swimming fry stage, when they must start foraging actively, at ~900 ° C degree days. Thus, starting with the recorded water temperature on 20 October each year (that is, from 1955 and onwards), the daily water temperatures were accumulated to predict the date of hatching and reaching the free-swimming stage in each year. However, to compensate for a slightly higher than expected development rate of eggs at low temperatures [59] , [60] , 1.2 ° C was first added to every day with water temperature <3 ° C (as recommended and used by commercial fish farmers in the region that rear eggs for hatching). The ordinal dates when 485, 750 and 900 degree days were reached were noted as the predicted dates for (i) hatching, (ii) partly consumed yolk sac and (iii) becoming actively foraging in a particular year, respectively. To analyse if winter water temperatures have a time-delayed effect on the stock of Arctic charr we correlated the estimated Julian day (ordinal date) for reaching the different fry stages in each year, with the normalized catch, up to eight years later. Here we present results based on the predicted dates for reaching the actively foraging free-swimming stage ( D Fx ) only, because it should be the abundance of resources at this time that is critical for the survival of the fry and thus for successful recruitment of great Arctic charr. Analyses on the other dates produced qualitatively similar, but statistically weaker relations. Zooplankton spring peak and degree of trophic mismatch Independent data on the variation in zooplankton abundance during spring in Lake Vättern is not available. However, there is now ample evidence of both timing and abundance of zooplankton being linked to climate [61] , [62] , [63] , [64] , [65] , [66] , [67] , implying that spring water temperature in Lake Vättern affects the timing of the peak in spring zooplankton. We made the reasonable assumption that the combination of time of spawning in the fall and development rate of eggs and larvae of great Arctic charr have evolved so that the date for reaching the free-swimming stage, on average and in the absence of current climate change, matches a period with abundant resources for the larvae. This implies that the mean date for reaching the actively foraging fry stage ( ), before significant winter warming occurred, could be used as a proxy for the expected pre-warming date for the spring peak in zooplankton ( ). Thus, we calculated the expected date for the zooplankton peak from the mean ordinal dates for reaching the fry stage during the years 1955–1988. During this period, there is no significant trend for this event nor for winter water temperature, while the following period is characterized by significant warming and an associated trend of advancing date for reaching the free-swimming stage ( Fig. 3 ). Thus, the date for spring peak in zooplankton in a particular year ( D Zx ) was estimated from the relationship: , where T Wx is the observed average spring (March) water temperature (° C) in year x , (=1.00 ° C) the mean average spring water temperature during 1955–1988, (=154) the mean (expected) Julian day (ordinal date) for the spring peak in zooplankton during 1955–1988, and k is the slope quantifying the response to water temperature, of the date for the spring peak in zooplankton. For the value of k (=−12), we consulted Burthe et al. [68] , who estimated the parameters of the linear relationship between zooplankton phenology and mean spring water temperature. To analyse if the survival of fry, and subsequently successful recruitment to the stock of arctic charr, is affected by the date for reaching the free-swimming stage of fry relative to the zooplankton peak, we developed an index that estimates the total trophic mismatch (Λ x ) between fry and their zooplankton prey that has affected the catch in year x , and was defined as the weighted mean of the trophic mismatches of all the age classes (here age classes 4 to 13) with a predicted proportional contribution ( p j , Supplementary Fig. 5a ) of more than 0.005 to the catch (that is, (where λ x−j is the degree of trophic mismatch for the fish that were fry in year x−j ). The normalized catch was then correlated with this index. The expected contributions of age classes of Arctic charr to the catch were calculated using estimated size selectivity curves for great Arctic charr [69] in gillnets with mesh sizes 35 and 43 mm (which are the mesh sizes used historically in the Arctic charr and whitefish fishery in Lake Vättern), in combination with a realistic age-frequency distribution in the stock (obtained from survey-based estimates of mortality rates in the population [46] and a size-at-age relationship, Supplementary Fig. 5b ). The degree of trophic mismatch ( λ x ) for fry in year x was defined as the difference between the estimated dates for fry emergence ( D Fx ) and the predicted date for spring peak in zooplankton ( D Zx ), that is, ). Statistical analyses Our analyses focuses on if (i) the date for reaching the actively foraging fry stage in spring, (ii) the availability of crustaceans and (iii) the availability of vendace have detectable effects on the stock of great Arctic charr in Lake Vättern, as measured by the normalized catches. To analyse if, and how, the associations between vendace and crustaceans on one hand and great Arctic charr on the other have changed over the study period, we analysed the correlation between time series data within short time intervals. Thus, the top–down and bottom–up ‘trophic control indices’ were (as in Litzow and Ciannelli [42] ) defined as the Pearson product moment correlation coefficient between consumer and resource time series, on a sliding time window. More specifically, for the bottom–up index, the detrended time series of charr was correlated to that of vendace 2 years earlier, and for the top–down index the detrended time series of charr was correlated to that of vendace 1 year later (because the cross-correlation between charr and vendace, Fig. 4b , showed a significant positive and negative correlation at a time lag of −2 and +1 respectively). Furthermore, to be able to detect short-term changes in association (trophic control), we used a narrow sliding time window of 3 years. A time window of 5 and 7 years produced qualitatively similar results, but was slightly less able to detect rapid changes in the association between charr and vendace. How to cite this article: Jonsson, T. and Setzer, M. A freshwater predator hit twice by effects of warming across trophic levels. Nat. Commun. 6:5992 doi: 10.1038/ncomms6992 (2015).